In vivoodourant response properties of migrating adult-born neurons in the mouse olfactory bulb Juxtaglomerular neurons (JGNs) of the mammalian olfactory bulb are generated throughout life. Their integration into the preexisting neural network, their differentiation and survival therein depend on sensory activity, but when and how these adult-born cells acquire responsiveness to sensory stimuli remains unknown. In vivo two-photon imaging of retrovirally labelled adult-born JGNs reveals that ~90% of the cells arrive at the glomerular layer after day post injection (DPI) 7. After arrival, adult-born JGNs are still migrating, but at DPI 9, 52% of them have odour-evoked Ca 2+ signals. Their odourant sensitivity closely resembles that of the parent glomerulus and surrounding JGNs, and their spontaneous and odour-evoked spiking is similar to that of their resident neighbours. Our data reveal a remarkably rapid functional integration of adult-born cells into the preexisting neural network. The mature pattern of odour-evoked responses of these cells strongly contrasts with their molecular phenotype, which is typical of immature, migrating neuroblasts. Throughout life, adult-born neurons integrate into the preexisting neural circuitry of the mammalian olfactory bulb (OB). Their progenitors are generated in the subependymal zone lining the walls of the lateral ventricles and in the rostral migratory stream (RMS), the route used by progenitors for migration towards the OB. Thousands of cells reach the OB every day [1] . The majority of them differentiate into granule cells (GCs) but some 5%–10% enter the glomerular layer of the bulb to become juxtaglomerular neurons (JGNs) [2] . In mice, there are 1.2 million JGNs [3] and the fraction of adult-born JGNs continuously increases with age reaching ≥30% in 9-month-old animals [4] . This is in contrast to the GC layer, in which the fraction of adult-born neurons is maintained at ~12% of cells throughout life. As 95% of adult-born cells are GABAergic interneurons (granule, periglomerular and short axon cells) and only 5% are glutamatergic short axon cells [5] , the addition of the adult-born neurons mostly translates into strengthening inhibition within the neural network of the OB. However, only ~50% of the GCs [6] and the JGNs [7] added to the OB during adulthood survive over prolonged periods of time. Our current knowledge about the maturation of adult-born cells in the OB is dominated by the data obtained in GCs. GCs reach their final maturation 4 weeks after birth, sequentially passing through five distinct maturation stages, from neuroblasts migrating in the RMS to mature GCs with a complex dendritic arbour [6] , [8] . During the third week after birth, adult-born GCs develop input synapses in their proximal dendritic domain [9] . Most of their dendro-dendritic output synapses develop only during the fourth week after birth. These data together with the ability to fire action potentials (APs), developing ~4 weeks after virus injection in the subependymal zone [10] , suggest that adult-born GCs have to listen to the neural network they integrate into for several weeks before they can send any output signals and thus influence the ongoing neuronal activity [11] , [12] . Recent studies re-visited this issue using optogenetics and lentiviral injections into the RMS (usually labelling 3- to 4-day-old neuroblasts on their way from the subependymal zone to the OB [13] ) and suggested that reliable spiking of adult-born GCs develops within <2 weeks post injection (wpi) [14] . The earliest functional GABAergic and glutamatergic synaptic inputs were found at day post injection (DPI) 3 (ref. 15 ). GABAergic synaptic inputs seemed to mature by DPI 7 (ref. 15 ), whereas the maturation of glutamatergic synaptic inputs was not completed before DPI 21 (ref. 10 ). Similar data were obtained for adult-born JGNs [16] . Here, GABAergic inputs appeared at DPI 4 and the first glutamatergic inputs were seen at DPI 7. However, mature glutamatergic synapses (that is, synapses with high AMPA (α-amino-3-hydroxy-5-methyl-4-isoxazolepropionic acid)/NMDA ( N -methyl- D -aspartate) ratio) were detected only from DPI 45 onwards [16] . Accumulating evidence suggests that adult-born neurons are critically important for the perceptual and memory functions of the OB such as odourant detection [17] , [18] (but see ref. 19 ), short- and long-term olfactory memory [17] , [19] , [20] , [21] , odourant discrimination [22] , [23] , [24] , [25] and learning an odour–reward association [21] . In addition, recent studies have suggested the involvement of adult-born neurons in innate olfactory responses including predator avoidance and sexual behaviours [26] , [27] , and olfactory fear conditioning [28] . By selectively expressing channelrhodopsin-2 in adult-born cells, Alonso et al . [25] has found that their light-induced activation accelerates odour discrimination learning in mice and improves the formation of olfactory memory. The authors have also shown that direct optogenetic activation of adult-born neurons selectively improved mice’s performance in a difficult but not in a simple odour-discrimination task. These observations imply an important role of adult-born neurons for the proper function of the olfactory system. Recent literature also emphasizes the role of extrinsic signals, such as odourant-induced activity, on the integration, fate determination and maintenance of adult-born cells [29] . For example, synaptogenesis in adult-born neurons was shown to occur in an activity-dependent manner. Sensory deprivation decreased the synaptic wiring of adult-born neurons [30] , [31] , whereas sensory enrichment accelerated the development of adult-born JGNs. Thus, immature (DPI 12–14) JGNs growing within sensory enriched loci had the morphological complexity of mature adult-born cells [32] . This was true for all of the tested morphological parameters, including total dendritic branch length, number of branch points, the number of PSD95-positive puncta per neuron (used by the authors as a proxy for synapses) and the neurons’ spatial territory coverage [32] . In contrast, sensory deprivation seemed to specifically reduce the dendritic length, spine density and the total number of newborn but not of preexisting GCs [30] . Moreover, odour enrichment promoted the rate of survival and the integration of adult-born neurons [20] , [33] (but see ref. 18 ), whereas odour deprivation decreased their survival [6] , [34] . The survival was furthermore enhanced both by perceptual [35] and associative [24] , [36] , [37] olfactory learning. Despite of the key role of odour-evoked activity for the integration and survival of adult-born neurons, the properties and the pattern of the earliest odour-evoked responses, as well as the developmental stage at which they become responsive to odour stimuli remain unclear. In this study we combine immunocytochemistry, in vivo electrophysiology and two-photon Ca 2+ imaging, to show that adult-born JGNs become odour responsive <48 h after their arrival at the glomerular layer and before they reach their final destination. By DPI 9, the amplitudes of odour-evoked Ca 2+ transients, the odourant sensitivity of adult-born cells and the frequencies of odour-evoked APs in these cells are largely similar to that of the neighbouring resident neurons. The mature appearance of odour-evoked responses of these cells strongly contrasts with their molecular phenotype, which is typical for immature, migrating neuroblasts. Early odour responsiveness of adult-born cells Adult-born neurons were labelled with eGFP (enhanced green fluorescent protein) via the injection of eGFP-encoding retroviruses into the RMS. A simultaneous injection of retroviruses and a thymidine analogue bromodeoxyuridine (BrdU; intraperitoneal (i.p.)) resulted in 92.6±3.0% of double-positive cells ( Supplementary Fig. 1 ), showing that under these experimental conditions DPI approximately equals the days after the cell’s birth. At the day of the experiment, both eGFP + and eGFP − juxtaglomerular cells were labelled with a small-molecule Ca 2+ indicator Fura-PE3, using the multi-cell bolus loading technique [38] . This enabled us to compare odour-evoked Ca 2+ transients of adult-born eGFP + cells and their eGFP − neighbours. To do so, we first identified odourant responding glomeruli at low spatial resolution [39] and then zoomed in to record odour-evoked Ca 2+ transients from identified neurons ( Fig. 1a ). Surprisingly, by 9 days following retroviral birth-dating (DPI 9) many adult-born cells were odour responsive ( Fig. 1b,e ). To ascertain whether recorded fluorescence changes indeed originate from eGFP + cells, we constructed high-resolution activity maps (frame subtractions) of the imaged area by averaging the frames recorded during the 2-s-long interval before and during odourant presentation and subtracting the two images from each other. We counted only those cells as odour responsive, which were clearly discernible on the activity map (for example, asterisk in Fig. 1c ). Using this criterion, we calculated the fraction of odour-responsive eGFP + cells at a given DPI by testing the responsiveness of all eGFP + cells that sent their dendrites into odour-responsive glomeruli (for example, Fig. 1a ). The results ( Fig. 1e , right) show that at DPI 9, 52.4% of adult-born cells already respond to olfactory stimuli, and that the fraction of responding cells reaches a plateau (~90%) at DPI 18–20. Next, we labelled adult-born cells with the novel genetically encoded ratiometric Ca 2+ indicator Twitch-2B [40] . In this case, clear odour-evoked Ca 2+ transients were recorded from both somata and dendrites of DPI 9 JGNs ( Fig. 1d ). In a good agreement with the data described above, 47.7% of the DPI 9 JGNs tested (31/65, n =4 mice) were odour responsive ( Fig. 1d,e , left). 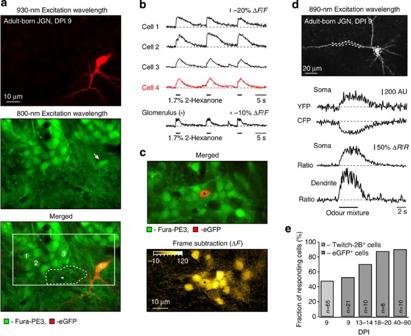Figure 1: Odour-evoked Ca2+transients in immature adult-born cells. (a) Top:in vivoimage of an eGFP+adult-born (DPI 9) juxtaglomerular cell located 60 μm below the dura imaged using 930 nm excitation light. Middle: the same area labelled with Fura-PE3 and imaged using 800 nm excitation light. The arrow points to the Fura-PE3-labelled eGFP+cell, as confirmed by the merged image (bottom). The solid rectangle in the bottom panel delineates the field of view chosen for the recordings inb. (b) Ca2+transients, evoked by three presentations of 2-hexanone in front of the mouse’s snout, recorded simultaneously from cells labelled by numbers ina(bottom) and from the parent glomerulus of the adult-born JGN (dotted outline and an asterisk). (c) Activity map-based identification of responding neurons in a different preparation. The top panel shows a merged image of Fura-PE3 and eGFP fluorescence recorded as illustrated ina. The bottom panel shows the activity map (frame subtraction, see Methods) for the same group of cells. The asterisk marks an eGFP+neuron. (d) Odour-evoked Ca2+signals (bottom) in an adult-born neuron (DPI 9) labelled with retrovirus encoding a FRET-based Ca2+indicator Twitch-2B (top). The cell was stimulated with a mixture of three odourants known to activate dorsal OB glomeruli (2-hexanone, isoamyl acetate and ethyl tiglate; 0.6% of saturated vapour each).Traces in the bottom panel illustrate somatic changes in fluorescence in both the yellow fluorescent protein (YFP) and cyan fluorescent protein (CFP) channels, as well as YFP/CFP ratio traces recorded from somatic and dendritic regions of interest shown in the upper image. (e) Bar graph summarizing the fraction of Twitch-2B+(left) and eGFP+(right) odour-responsive adult-born JGNs as a function of their age. The numbers of cells tested are given within each bar. Note that there is no significant difference between values obtained for DPI 9 cells with the two different calcium sensors (Pearson’sχ2-test,P=0.8). Figure 1: Odour-evoked Ca 2+ transients in immature adult-born cells. ( a ) Top: in vivo image of an eGFP + adult-born (DPI 9) juxtaglomerular cell located 60 μm below the dura imaged using 930 nm excitation light. Middle: the same area labelled with Fura-PE3 and imaged using 800 nm excitation light. The arrow points to the Fura-PE3-labelled eGFP + cell, as confirmed by the merged image (bottom). The solid rectangle in the bottom panel delineates the field of view chosen for the recordings in b . ( b ) Ca 2+ transients, evoked by three presentations of 2-hexanone in front of the mouse’s snout, recorded simultaneously from cells labelled by numbers in a (bottom) and from the parent glomerulus of the adult-born JGN (dotted outline and an asterisk). ( c ) Activity map-based identification of responding neurons in a different preparation. The top panel shows a merged image of Fura-PE3 and eGFP fluorescence recorded as illustrated in a . The bottom panel shows the activity map (frame subtraction, see Methods) for the same group of cells. The asterisk marks an eGFP + neuron. ( d ) Odour-evoked Ca 2+ signals (bottom) in an adult-born neuron (DPI 9) labelled with retrovirus encoding a FRET-based Ca 2+ indicator Twitch-2B (top). The cell was stimulated with a mixture of three odourants known to activate dorsal OB glomeruli (2-hexanone, isoamyl acetate and ethyl tiglate; 0.6% of saturated vapour each).Traces in the bottom panel illustrate somatic changes in fluorescence in both the yellow fluorescent protein (YFP) and cyan fluorescent protein (CFP) channels, as well as YFP/CFP ratio traces recorded from somatic and dendritic regions of interest shown in the upper image. ( e ) Bar graph summarizing the fraction of Twitch-2B + (left) and eGFP + (right) odour-responsive adult-born JGNs as a function of their age. The numbers of cells tested are given within each bar. Note that there is no significant difference between values obtained for DPI 9 cells with the two different calcium sensors (Pearson’s χ 2 -test, P =0.8). Full size image Odour-evoked responses in migrating cells When imaging the same adult-born JGNs over several hours, we realized that at DPI 9 many cells move within the field of view (for example, one cell in the middle (asterisk in the cell body) and another in the lower right corner of Fig. 2a ). When tested for odour-evoked responses for the first time, the migrating cell labelled with an asterisk was non-responding (upper panel in Fig. 2b and left panel in Fig. 2c ). However, it became responsive only 90 min later (lower panel in Fig. 2b and right panel in Fig. 2c ). Note that the general odour responsiveness of the surrounding cells was not substantially changed between the two trials ( Fig. 2d,e ). Similar observations were made for four additional adult-born cells. 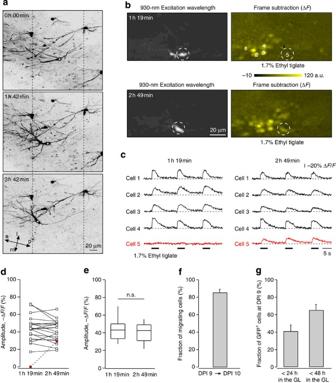Figure 2: Rapid appearance of odour-evoked responses in migrating cells. (a) Images of a group of adult-born JGNs taken at DPI 9. Each image is a maximum intensity projection of a stack of images (0–90 μm depth and 1 μm step) taken at different time points as indicated (see timestamp and relative time). The migrating neuron in the middle of the field of view is labelled with an asterisk. The arrows in the lower left corner indicate the orientation of this plane of view within the bulb (a–p, anterior–posterior; l–m, lateral–medial). Broken lines are reference lines attached to immobile cells. (b) Left: images of an eGFP+cell at two different time points (see timestamps) taken using 930 nm excitation light. Each image is an average of 12 consecutive image frames. Right: corresponding activity maps (frame subtraction, see Methods) recorded from the same field of view. Cells 1–4 are eGFP−neurons, cell 5 is the same neuron as the one labelled with an asterisk ina. (c) Responses of eGFP−cells 1–4 and the adult-born cell 5 (as marked inb) to three 4-s-long presentations of 1.7% ethyl tiglate at the two different time points (as indicated). (d) Amplitudes of odour-evoked Ca2+signals of all eGFP−cells that can be unequivocally distinguished within the imaging frame inb(white squares,n=20) as well as the migrating cell (red squares, cell 5 inc) recorded during the two consecutive trials illustrated inb. Note that change in the amplitude of migrating cell is larger than any other amplitude change observed in this experiment. (e) Box plots illustrating the distributions of response amplitudes of eGFP−cells ind. The two distributions are not significantly different (P=0.11, Wilcoxon signed-rank test). (f) Bar graph illustrating the fraction of migrating JGNs at DPI 9 (n=120 cells, 13 imaged areas, 3 mice). (g) Bar graph illustrating the distribution of age of cells imaged at DPI 9 in the glomerular layer (the same data set as inf). Figure 2: Rapid appearance of odour-evoked responses in migrating cells. ( a ) Images of a group of adult-born JGNs taken at DPI 9. Each image is a maximum intensity projection of a stack of images (0–90 μm depth and 1 μm step) taken at different time points as indicated (see timestamp and relative time). The migrating neuron in the middle of the field of view is labelled with an asterisk. The arrows in the lower left corner indicate the orientation of this plane of view within the bulb (a–p, anterior–posterior; l–m, lateral–medial). Broken lines are reference lines attached to immobile cells. ( b ) Left: images of an eGFP + cell at two different time points (see timestamps) taken using 930 nm excitation light. Each image is an average of 12 consecutive image frames. Right: corresponding activity maps (frame subtraction, see Methods) recorded from the same field of view. Cells 1–4 are eGFP − neurons, cell 5 is the same neuron as the one labelled with an asterisk in a . ( c ) Responses of eGFP − cells 1–4 and the adult-born cell 5 (as marked in b ) to three 4-s-long presentations of 1.7% ethyl tiglate at the two different time points (as indicated). ( d ) Amplitudes of odour-evoked Ca 2+ signals of all eGFP − cells that can be unequivocally distinguished within the imaging frame in b (white squares, n =20) as well as the migrating cell (red squares, cell 5 in c ) recorded during the two consecutive trials illustrated in b . Note that change in the amplitude of migrating cell is larger than any other amplitude change observed in this experiment. ( e ) Box plots illustrating the distributions of response amplitudes of eGFP − cells in d . The two distributions are not significantly different ( P =0.11, Wilcoxon signed-rank test). ( f ) Bar graph illustrating the fraction of migrating JGNs at DPI 9 ( n =120 cells, 13 imaged areas, 3 mice). ( g ) Bar graph illustrating the distribution of age of cells imaged at DPI 9 in the glomerular layer (the same data set as in f ). Full size image To estimate the fraction of cells migrating at DPI 9, we performed chronic imaging experiments and imaged the adult-born cells twice per day through an implanted cranial window [41] . Simultaneous blood vessel imaging ( Supplementary Fig. 2 ) was employed in each experiment to align the image fields across imaging sessions. Out of 120 cells ( n =13 imaging frames, 3 mice) sampled at DPI 9, 85.4% changed their location within the next 24 h ( Fig. 2f and Supplementary Fig. 2b ) and all of the cells changed location between DPI 9 and DPI 30. For 22 migrating cells, it was possible to precisely identify the location of their somata 12 and 24 h later (that is, at DPI 9.5 and DPI 10), and thus to calculate the distance they travelled between DPI 9 and DPI 10. This distance ranged from 8 to 163 μm (median 40.4 μm, n =22). Next, we estimated when the cells sampled at DPI 9 arrived at the glomerular layer. Although occasionally adult-born cells were already seen in the glomerular layer at DPI 5 or 6, the fraction of these early arriving cells was extremely low (<5%, Supplementary Fig. 2c ). Of the aforementioned 120 cells sampled at DPI 9, 64.8% were not present in the glomerular layer at DPI 7 and 40.7% arrived after the imaging session at DPI 8 ( Fig. 2g ). We conclude that adult-born cells start responding to odourants while migrating and before reaching their final destination within the glomerular layer. Moreover, the majority of the cells acquire the ability to respond to sensory stimuli in <48 h after entering the glomerular layer. Odourant response properties of immature adult-born neurons We first determined the odourant sensitivity of immature adult-born neurons. To obtain dose–response relationships for adult-born neurons and their parent glomeruli (that is, glomeruli they send their dendrites into, Fig. 3a ) we presented odourants at different concentrations (0.1%–9% of saturated vapour) in front of the mouse’s snout. Control experiments ensured that the Ca 2+ indicator dye was not saturated even at high odourant concentrations (9% of saturated vapour), because much larger Ca 2+ transients were evoked in these cells by local glutamate applications ( Supplementary Fig. 3 ). Surprisingly, already at DPI 9, adult-born JGNs responded with large Ca 2+ transients to low odourant concentrations (for example, see Fig. 3a,e ). In general, the relationship between odour concentration and response amplitude of the immature adult-born cells was very similar to that of their parent glomeruli ( Fig. 3a–d ), but differed significantly from that of other glomeruli within the field of view, which responded to the same odourant ( Fig. 3d ). It should be mentioned that glomerular signals recorded here are mixed signals comprising signals from presynaptic axons and their terminals, as well as postsynaptic cells projecting to this glomerulus. Presynaptic structures contribute ~60% of the amplitude of odour-evoked glomerular Ca 2+ signals and the remainder reflects the contribution of postsynaptic cells (see Fig. 2c in ref. 39 ). As odour-responsive cells surrounding odour-responsive glomeruli probably belong to the same functional unit [39] , we compared the amplitudes of odour-evoked Ca 2+ transients in adult-born JGNs (DPI 9) and the eGFP − neighbours. The maturity of eGFP − cells was proven by the fact that 98.0±0.4% of them were positive for markers of mature neurons (calbindin, calretinin, tyrosine hydroxylase (TH) or NeuN [7] ) and negative for the marker of immature neurons doublecortin (DCX; Supplementary Fig. 4 ). As DCX expression is present in the adult-born cells during the first 3 weeks of their life [16] , [42] , these data suggest that only 2% of eGFP − cells in our experiments are less than 3 weeks old. We found that for both eGFP + and eGFP − cells, the amplitudes of odour-evoked Ca 2+ transients were largely similar ( Fig. 3e ). A significant difference between the two could only be detected at the low odourant concentration (0.2% of saturated vapour). In a very few cases, we also saw an inhibited response to an odourant in an adult-born cell at DPI 9 ( n =2, an example is shown in Supplementary Fig. 5 ). As it is very likely to be that an inhibited response is generated within the glomerular circuitry [39] , this finding suggests an early and rather complex synaptic integration of these adult-born neurons. 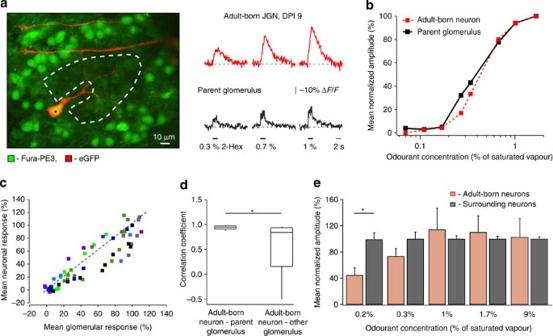Figure 3: Odourant-sensitivity of DPI 9 cells resembles that of the parent glomeruli. (a) Left panel: an image of an adult-born eGFP+neuron (asterisk) with dendrites in the parent glomerulus. The glomerulus is surrounded by numerous eGFP−JGNs stained with Fura-PE3. Right panel: representative Ca2+transients measured simultaneously from the soma of the adult-born cell (upper row) and the parent glomerulus (lower row; region of interest indicated by the dotted line) in response to 2-s-long presentations of 2-hexanone at three different concentrations (0.3%, 0.7% and 1% of saturated vapour). (b) Dose–response curves illustrating the amplitudes of Ca2+transients measured from the adult-born neuron (red) and the parent glomerulus (black) shown ina. The amplitudes were averaged across three to four trials and normalized to the maximal value measured at 1.7% of saturated vapour. (c) Pooled data from seven experiments similar to the one shown inaandb. The normalized amplitudes of odour-evoked responses of adult-born cells were plotted against that of their parent glomeruli. Each cell–glomerulus pair is shown in a different colour. The dotted line represents the linear least-squares fit of the data; the slope of the line is 1.04. (d) Pearson’s correlation coefficients of the response amplitudes for adult-born cell—parent glomerulus pairs (left,n=7) in comparison with the correlation coefficients between the amplitude of the adult-born cell response and that of other odour-responsive glomeruli located nearby (right,n=5). The two values are significantly different (P=0.04, Mann–Whitney test). (e) Comparison of mean amplitudes recorded pairwise from adult-born eGFP+cells (red,n=7) and surrounding eGFP−neurons (n=54) as a function of the odourant concentration. In each experiment and for each odourant concentration, the amplitudes of odour-evoked responses of individual cells were normalized to the mean value, calculated over the entire population of responding eGFP-negative cells. Note the significantly smaller mean response amplitude of the adult-born JGNs at the 0.2% of saturated vapour (P<0.05, pairedt-test with the Bonferroni correction for multiple comparisons). All adult-born cells analysed ina–ewere DPI 9. Figure 3: Odourant-sensitivity of DPI 9 cells resembles that of the parent glomeruli. ( a ) Left panel: an image of an adult-born eGFP + neuron (asterisk) with dendrites in the parent glomerulus. The glomerulus is surrounded by numerous eGFP − JGNs stained with Fura-PE3. Right panel: representative Ca 2+ transients measured simultaneously from the soma of the adult-born cell (upper row) and the parent glomerulus (lower row; region of interest indicated by the dotted line) in response to 2-s-long presentations of 2-hexanone at three different concentrations (0.3%, 0.7% and 1% of saturated vapour). ( b ) Dose–response curves illustrating the amplitudes of Ca 2+ transients measured from the adult-born neuron (red) and the parent glomerulus (black) shown in a . The amplitudes were averaged across three to four trials and normalized to the maximal value measured at 1.7% of saturated vapour. ( c ) Pooled data from seven experiments similar to the one shown in a and b . The normalized amplitudes of odour-evoked responses of adult-born cells were plotted against that of their parent glomeruli. Each cell–glomerulus pair is shown in a different colour. The dotted line represents the linear least-squares fit of the data; the slope of the line is 1.04. ( d ) Pearson’s correlation coefficients of the response amplitudes for adult-born cell—parent glomerulus pairs (left, n =7) in comparison with the correlation coefficients between the amplitude of the adult-born cell response and that of other odour-responsive glomeruli located nearby (right, n =5). The two values are significantly different ( P =0.04, Mann–Whitney test). ( e ) Comparison of mean amplitudes recorded pairwise from adult-born eGFP + cells (red, n =7) and surrounding eGFP − neurons ( n =54) as a function of the odourant concentration. In each experiment and for each odourant concentration, the amplitudes of odour-evoked responses of individual cells were normalized to the mean value, calculated over the entire population of responding eGFP-negative cells. Note the significantly smaller mean response amplitude of the adult-born JGNs at the 0.2% of saturated vapour ( P <0.05, paired t -test with the Bonferroni correction for multiple comparisons). All adult-born cells analysed in a – e were DPI 9. Full size image In acute tissue slices, glutamatergic synapses on immature adult-born JGNs are characterized by a relative predominance of NMDA over AMPA receptors [16] . We tested whether the odour-evoked Ca 2+ transients in eGFP + DPI 9 cells were more sensitive to NMDA receptor blocker CGP-37849 compared with odour-evoked Ca 2+ transients in surrounding eGFP − cells. An ~40-min-long topical application of CGP-37849 to the surface of the OB (see Methods) resulted in a significant and reversible decrease of the amplitude and the area under the Ca 2+ transients in both eGFP + and eGFP − cells ( Fig. 4 ). Of note, the degree of blockade varied between individual eGFP − cells in the same experiment ( Fig. 4a ). On average, however, there was no significant difference between the eGFP + and eGFP − cells for both parameters tested ( P >0.05, Wilcoxon signed-rank test; Fig. 4b,c ). Addition of the AMPA receptor blocker CNQX (50 μM) to the CGP-37849 containing solution further inhibited odour-evoked Ca 2+ transients (median normalized amplitude of odour-evoked Ca 2+ transients was 24% of the control value for eGFP − ( n =54 cells, 5 mice) and 10% for eGFP + DPI 9 cells ( n =5 cells, 5 mice)), suggesting that the latter strongly rely on activation of glutamate receptors ( Fig. 4b,c ). Taken together, the above data suggest that shortly after arrival of adult-born JGNs at the glomerular layer, the odour-evoked Ca 2+ transients in these cells have properties largely similar to those of their mature neighbours. 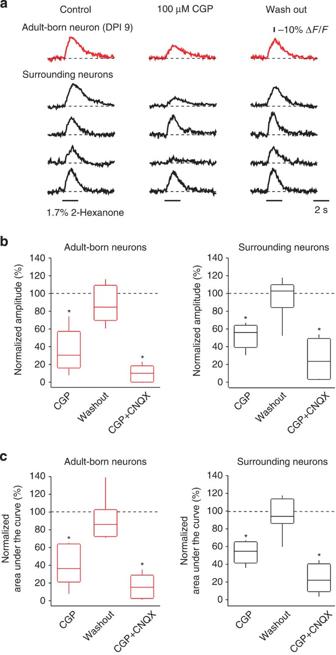Figure 4: Contribution of glutamate receptors to odour-evoked Ca2+transients in adult-born cells. (a) A representative experiment (repeated eight times in total, see below) illustrating odour-evoked Ca2+transients of an adult-born JGN (DPI 9, red traces) and four neighbouring eGFP−neurons (black traces). Each transient is an average of three consecutive trials recorded under control conditions (left), in the presence of the NMDA receptor blocker CGP (middle) and after washout of CGP (right). CGP was added to the chamber-perfusing solution for 45 min and washed out for 55 min before recording the ‘washout’ data. (b,c) Box plots summarizing the effects of CGP (100 μM) and AMPA receptor blocker CNQX (50 μM) on the normalized amplitudes of odour-evoked Ca2+transients (b) and normalized areas under the Ca2+transients (c). For CGP,n=8 eGFP+DPI 9 JGNs (red bars) andn=103 neighbouring eGFP−neurons from 8 experiments (black bars). The washout of CGP took 45–90 min. For subsequent application of the mixture of CGP (100 μM) and CNQX (50 μM),n=5 DPI 9 JGNs and 54 neighbouring eGFP−neurons from 5 experiments. Asterisks denote significant differences between the data obtained in control and in the presence of the drugs (P≤0.01, Wilcoxon signed-rank test). For CGP and CNQX+CGP, there was no significant difference between data obtained from eGFP+and eGFP−cells (P≥0.05, Wilcoxon signed-rank test). Figure 4: Contribution of glutamate receptors to odour-evoked Ca 2+ transients in adult-born cells. ( a ) A representative experiment (repeated eight times in total, see below) illustrating odour-evoked Ca 2+ transients of an adult-born JGN (DPI 9, red traces) and four neighbouring eGFP − neurons (black traces). Each transient is an average of three consecutive trials recorded under control conditions (left), in the presence of the NMDA receptor blocker CGP (middle) and after washout of CGP (right). CGP was added to the chamber-perfusing solution for 45 min and washed out for 55 min before recording the ‘washout’ data. ( b , c ) Box plots summarizing the effects of CGP (100 μM) and AMPA receptor blocker CNQX (50 μM) on the normalized amplitudes of odour-evoked Ca 2+ transients ( b ) and normalized areas under the Ca 2+ transients ( c ). For CGP, n =8 eGFP + DPI 9 JGNs (red bars) and n =103 neighbouring eGFP − neurons from 8 experiments (black bars). The washout of CGP took 45–90 min. For subsequent application of the mixture of CGP (100 μM) and CNQX (50 μM), n =5 DPI 9 JGNs and 54 neighbouring eGFP − neurons from 5 experiments. Asterisks denote significant differences between the data obtained in control and in the presence of the drugs ( P ≤0.01, Wilcoxon signed-rank test). For CGP and CNQX+CGP, there was no significant difference between data obtained from eGFP + and eGFP − cells ( P ≥0.05, Wilcoxon signed-rank test). Full size image To characterize the AP firing of immature adult-born JGNs, we performed targeted loose-patch recordings from odour-responsive cells. At DPI 9–11, 88.3% of the cells ( n =12) fired APs in the absence of odourants ( Fig. 5a ), but the frequency of AP firing was low, significantly lower than the background spike frequency in DPI 50–90 cells ( Fig. 5d ). 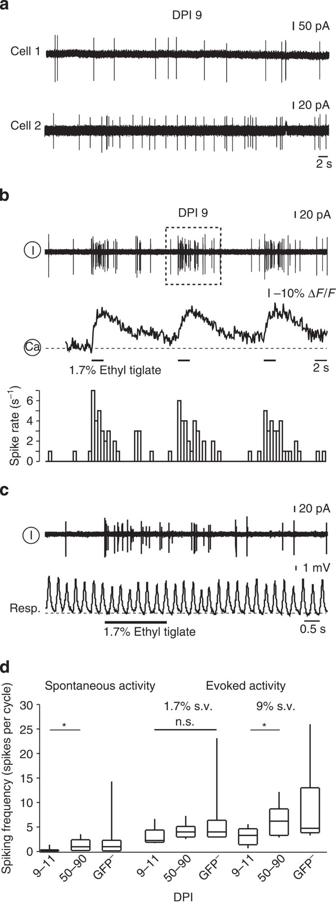Figure 5: Spontaneous and odour-evoked AP firing of adult-born cells. (a) Examples of the background AP firing recorded at DPI 9 from two adult-born JGNs in a loose-seal cell-attached configuration. (b) Simultaneous Ca2+imaging and loose-seal cell-attached recordings from an adult-born cell (DPI 9). The top trace is the electrical recording, the middle trace is the calcium signal and the bottom trace is the peristimulus time histogram obtained in the same trial (bin width=500 ms). (c) The boxed region inbis shown on an expanded time scale together with the respiration trace. Positive deflection of the respiration signal (lower trace, Resp.) corresponds to the inhalation phase. (d) Box plot summarizing spiking properties of adult-born JGNs measured under two different conditions: at rest (Spontaneous activity) and during the application of different odourant concentrations (1.7% and 9% of saturated vapour, Evoked activity). Recordings were made from three populations of juxtaglomerular cells: immature adult-born eGFP+cells (DPI 9–11), mature adult-born eGFP+cells (DPI 50–90) and eGFP−cells. From left to right,n=7, 12, 14, 6, 9, 13, 5, 11 and 7 cells. Asterisks denote significant differences between the groups (P<0.05, Welch’sU-test and Mann–Whitney test). All cells tested showed odour-evoked Ca2+signals. Figure 5: Spontaneous and odour-evoked AP firing of adult-born cells. ( a ) Examples of the background AP firing recorded at DPI 9 from two adult-born JGNs in a loose-seal cell-attached configuration. ( b ) Simultaneous Ca 2+ imaging and loose-seal cell-attached recordings from an adult-born cell (DPI 9). The top trace is the electrical recording, the middle trace is the calcium signal and the bottom trace is the peristimulus time histogram obtained in the same trial (bin width=500 ms). ( c ) The boxed region in b is shown on an expanded time scale together with the respiration trace. Positive deflection of the respiration signal (lower trace, Resp.) corresponds to the inhalation phase. ( d ) Box plot summarizing spiking properties of adult-born JGNs measured under two different conditions: at rest (Spontaneous activity) and during the application of different odourant concentrations (1.7% and 9% of saturated vapour, Evoked activity). Recordings were made from three populations of juxtaglomerular cells: immature adult-born eGFP + cells (DPI 9–11), mature adult-born eGFP + cells (DPI 50–90) and eGFP − cells. From left to right, n =7, 12, 14, 6, 9, 13, 5, 11 and 7 cells. Asterisks denote significant differences between the groups ( P <0.05, Welch’s U -test and Mann–Whitney test). All cells tested showed odour-evoked Ca 2+ signals. Full size image To test for age-dependent changes of spiking properties within the group of DPI 50–90 cells, we split this population into two subgroups (DPI 50–60 and DPI 70–90). We have not observed any significant difference between the spontaneous ( n =5 and 7, P =0.26, Welch’s U -test) and odour-evoked (see below; n =4 and 5, P =0.96 for 1.7% of s.v. and n =5 and 6, P =0.68 for 9% of s.v., Welch’s U -test) spiking frequencies of these cells. Therefore, the data from all DPI 50–90 cells were lumped together. On application of an odourant we observed an increase in the AP frequency of DPI 9 cells parallelled by an increase in the intracellular free Ca 2+ concentration ([Ca 2+ ] i ; Fig. 5b ). At physiologically relevant odourant concentrations (for example, 1.7% of saturated vapour), the magnitude of odour-evoked responses of immature (DPI 9–11) adult-born JGNs was similar to that of mature (DPI 50–90) and eGFP − cells ( Fig. 5d ). At high odourant concentrations (9% of saturated vapour), the significant difference in response magnitude was only observed between DPI 9–11 and DPI 50–90 cells, suggesting that DPI 50–90 cells are able to fire at higher maximal frequencies compared with immature adult-born JGNs. Consistent with data shown in Fig. 3e , we did not observe any significant difference between DPI 9–11 and surrounding GFP − cells at 9% of saturated vapour. Moreover, we did not observe any difference between the two age groups of adult-born JGNs when comparing the timing of AP firing during the respiratory cycle (as determined by the method of mean vector analysis, see Methods). The fraction of cells whose firing was phase locked during the odourant (1.7% of saturated vapour) presentation was 66.7% (4/6 cells) at DPI 9 and 55.6% (5/9 cells) at DPI 50–90. The mean phases of phase-locked cells were 225° and 201°, respectively ( P =0.4, Student’s t -test). Thus, at physiological odourant concentrations, odour-evoked AP firing of immature adult-born JGNs closely mimic that of mature adult-born neurons in respect to both response magnitude and phase tuning. Taken together, Ca 2+ imaging, pharmacological and electrophysiological data, all suggest that in vivo odourant response properties of adult-born DPI 9 JGNs resemble that of their mature neighbours. Putative output synapses of immature adult-born neurons As immature adult-born JGNs at DPI 9 respond to odourant stimulation with APs accompanied by large somatic and dendritic Ca 2+ transients, we wondered whether these inputs would result in synaptic output. Therefore, we labelled the cells with a marker for GABAergic presynaptic specializations VGAT (the vesicular γ-aminobutyric acid transporter). As expected [43] , this resulted in punctate labelling of the OB tissue. Some of these puncta were found inside the eGFP + adult-born JGNs ( Fig. 6a,b ). At DPI 9, 43.9% of adult-born neurons were VGAT positive ( n =55 cells in 5 mice, Fig. 6c ). However, only a few (one to five) VGAT-positive puncta were found in each positive cell. The number of VGAT-positive puncta increased significantly as the cells matured ( Fig. 6d ). The presence of molecular markers of vesicular release of GABA in adult-born neurons as early as DPI 9 suggests that these cells might be able to inhibit other cells within the circuitry by means of activity-dependent GABA release. 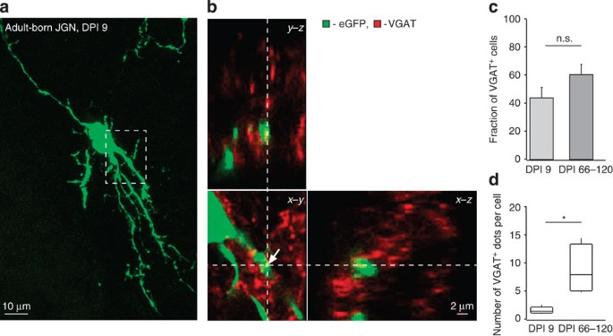Figure 6: GABAergic outputs of adult-born juxtaglomerular cells. (a) Maximum-intensity projection image of the stack of 67 confocal image planes spaced by 0.45 μm. The cell shown is an adult-born JGN at DPI 9 double-stained for eGFP (green) and VGAT (red). (b) Single confocal plane image (x–y) of the area delineated by a broken line ina. An arrow points to a VGAT-positive dot located within an eGFP-positive dendrite. The same dot can be visualized in the orthogonalx–zandy–zprojections using broken lines as landmarks. (c) Bar graph illustrating the fraction of VGAT-positive adult-born cells at DPI 9 (n=55 cells from 5 mice) and DPI 66–120 (70 cells, 4 mice), respectively (P=0.15, Student’st-test). (d) Box plot illustrating the number of VGAT-positive dots (that is, presumptive GABA release sites) per cell in the same two age groups (P<0.05, Mann–Whitney test). Figure 6: GABAergic outputs of adult-born juxtaglomerular cells. ( a ) Maximum-intensity projection image of the stack of 67 confocal image planes spaced by 0.45 μm. The cell shown is an adult-born JGN at DPI 9 double-stained for eGFP (green) and VGAT (red). ( b ) Single confocal plane image ( x – y ) of the area delineated by a broken line in a . An arrow points to a VGAT-positive dot located within an eGFP-positive dendrite. The same dot can be visualized in the orthogonal x – z and y – z projections using broken lines as landmarks. ( c ) Bar graph illustrating the fraction of VGAT-positive adult-born cells at DPI 9 ( n =55 cells from 5 mice) and DPI 66–120 (70 cells, 4 mice), respectively ( P =0.15, Student’s t -test). ( d ) Box plot illustrating the number of VGAT-positive dots (that is, presumptive GABA release sites) per cell in the same two age groups ( P <0.05, Mann–Whitney test). Full size image Chemical properties of immature adult-born neurons Taking into account rapid maturation of functional properties of adult-born cells, we tested whether their molecular phenotype matures at the same pace. As mature adult-born JGNs are known to express different subtype-specific markers (see above), we tested whether these markers were already expressed at DPI 9 ( Supplementary Fig. 6 ). The expression of these marker proteins was extremely limited at DPI 9. Immature adult-born JGNs were almost completely negative for TH and calbindin, and only 10.6±1.9% of cells tested ( n =152 cells in 5 mice) were positive for calretinin ( Supplementary Fig. 6c , left). Consistent with their immature molecular phenotype and migrating behaviour, all cells were positive for DCX and 93.2±1.5% of the cells were positive for the Polysialic acid neural cell adhesion molecule (PSA-NCAM) ( n =109 cells in 4 mice), resembling, in this respect, migrating neuroblasts [1] , [44] . When tested at 20–24 DPI, 26.4%, 27.3% and 7.7% of adult-born JGNs were positive for TH, calretinin and calbindin, respectively ( Supplementary Fig. 6c , middle). These data were largely consistent with data obtained by others at 30 DPI [7] , [45] . At 120 DPI, the fractions of TH-, calretinin- and calbindin-positive cells were 17.4%, 37.6% and 16.2%, respectively ( Supplementary Fig. 6c , right). Thus, in contrast to an extremely fast maturation of their odour-response properties, the molecular phenotypes of adult-born JGNs mature at a much slower pace. To our knowledge, this is the first in vivo study analysing functional properties of migrating adult-born cells. Our conservative estimates suggest that as early as 48 h after their arrival at the glomerular layer of the OB, these cells fire spontaneous and odourant-evoked APs, and respond to physiologically relevant sensory stimuli with large transient increases in [Ca 2+ ] i . These findings are in contrast to what could be inferred from previous in vitro data (see below). In addition, they suggest that unlike the initial assembly of neural circuits, which is mostly driven by intrinsic, spontaneous activity (for a review, see, for example, ref. 46 ), the integration of immature adult-born cells can additionally rely on extrinsic, sensory-driven signals. Our results show that the odour responsiveness of JGNs at DPI 9 is very similar to that of mature cells. Thus, 9 days after birth, adult-born JGNs respond to odourant concentrations as low as 0.2% of saturated vapour, have odourant response properties similar to that of their parent glomeruli and largely similar to that of neighbouring mature JGNs. A significant difference in the amplitudes of odour-evoked Ca 2+ transients between DPI 9 adult-born and surrounding mature neurons was observed only at very-low odourant concentrations. These in vivo data imply that intrabulbar connectivity of adult-born JGNs develops much faster than suggested by the previous in vitro data. In vitro , in the lentivirus-stained adult-born JGNs (which are usually 3–4 days older than the cells studied here (compare ref. 10 with ref. 14 )), the first glutamatergic synaptic inputs were seen at DPI 7 (ref. 16 ), corresponding to DPI 10–11 in our experiments. However, in our in vivo measurements we found large suprathreshold odour-evoked responses, mediated by glutamatergic synapses at DPI 9. Previous in vitro data have also highlighted a specific role of NMDA receptors for functional signalling of immature adult-born neurons. There is, for example, more than a twofold difference between the AMPA/NMDA receptor ratio at olfactory nerve synapses for excitatory postsynaptic currents of mature and immature adult-born JGNs [16] . Moreover, immature adult-born GCs were shown to have a depolarized resting membrane potential (favouring the activation of NMDA receptors) and NMDA receptor-dependent formation/retraction of filopodia on distal dendrites [10] , [47] . Consistently, our in vivo data show that odour-evoked Ca 2+ transients of immature adult-born JGNs contain a large NMDA receptor-mediated component. However, the contribution of NMDA receptors to odour-evoked Ca 2+ transients of mature eGFP − cells is similar. These data suggest that odour processing by JGNs depends on activation of NMDA receptors at any age and the correct pharmacological profile of odour-evoked Ca 2+ transients in these cells is acquired by DPI 9. This unusually strong recruitment of NMDA receptors during sensory signalling of JGNs is most probably due to the fact that sensory stimuli often evoke barrages of excitatory postsynaptic potentials accompanied by a burst of APs (see, for example, ref. 39 ), which are capable of depolarizing the cell and removing the Mg 2+ block of NMDA receptors. Alternatively, some NMDA receptors might be activated due to intraglomerular glutamate spillover, known to depolarize mature periglomerular cells during synchronized mitral cell activity [48] , [49] . Almost 90% of odour-responsive immature JGNs fired spontaneous APs, suggesting that in these adult-born cells the ability to spike develops before DPI 9. These data are at odds with the earlier data of Carleton et al . [10] obtained for adult-born GCs, but is more consistent with recent in vitro data [14] , [16] . In vivo , however, the synaptic connectivity of DPI 9 cells is strong enough to elicit suprathreshold EPSPs even at rest, whereas in slices the cells of the similar age just gain the ability to fire APs in response to current injections [16] . In general, the spontaneous spike rate of DPI 9–11 cells was significantly lower than that of mature DPI 50–90 neurons. However, we have observed two cells with inhibited odourant responses that probably fired at much higher frequencies (for example, cell 1 in Supplementary Fig. 5 ). To have an inhibited calcium response to an odourant, the cell had to continuously fire at rest (as evidenced by the high resting yellow fluorescent protein/cyan fluorescent protein ratio of this cell). Although the incidence of DPI 9 cells with inhibited responses was too low for targeted loose-patch recordings, our previous data [39] suggest that spiking frequencies of such cells are at least comparable with those of DPI 50–90 neurons. In line with our imaging data, the frequency of odourant-evoked APs was similar between immature and mature adult-born neurons and their eGFP − neighbours at physiological odourant concentrations (for example, 1.7% of saturated vapour). As expected for AP-induced Ca 2+ transients, odour-evoked signals invaded not only the soma of the cell but also its dendritic compartments. As was shown previously [50] , such dendritic Ca 2+ signals are required for activity-dependent release of GABA from dendrites of periglomerular cells. Remarkably, our data suggest that morphological correlates of GABAergic output synapses are present at adult-born JGNs as early as 9 days after their birth. This is ~1 week earlier than suggested by previous results [14] , [45] . However, in line with the previous studies, the number of presumed output synapses per adult-born JGN was low at 9 DPI and increased significantly as the adult-born cells matured. Thus, although functionally mature input signals are likely to be capable of generating some synaptic output as early as DPI 9, the latter is likely to be immature. Does the similarity of odourant response properties between DPI 9 cells and their GFP − neighbours suggest that DPI 9 cells are fully mature? Clearly not. First, DPI 9 cells express molecular markers of immature migrating neuroblasts and are negative for markers of mature neurons. Second, their background spiking frequency as well as their responses to very low odourant concentrations differ from that of older, more mature neurons. These data are consistent with the assumption that the density of synaptic inputs onto DPI 9 cells is sparse, but this sparseness is compensated for by their increased ability to depolarize the cell, probably due to a high input resistance [16] and/or increased excitability [51] of the adult-born cells. Third, DPI 9 cells contain very few putative output synapses, significantly less than mature adult-born neurons. Moreover, in contrast to the later developmental stage (8–9 wpi of lentivirus), when adult-born neurons sample information from glomeruli located up to 450 μm apart [45] , DPI 9 cells seem to rely on information provided by the immediately adjacent glomeruli. Interestingly, our data show that compared with DPI 9 cells DPI 50–90 neurons are able to respond with significantly higher firing rates to high odourant concentrations. This is in line with a recent paper [45] , which studied in vivo spiking properties of adult-born JGNs at 2 and 4 wpi (comparable to DPI 18 and 32 of the present study). The data of Livneh et al . [45] suggest that the frequency of odourant-evoked AP firing is highest and the odourant selectivity is lowest at 4 wpi (see Fig. 3 of ref. 45 ). Therefore, 4 wpi neurons are more easily recruited by odour stimulation. Together with our study, these data reveal a bell-shaped developmental profile for some of the odour-response parameters of adult-born neurons (for example, the frequency of odourant-evoked AP firing), while others (for example, spontaneous and odour-evoked respiration phase tuning) seem to remain constant throughout development. Surprisingly, the mature-like odour-evoked input signals encountered at DPI 9 were found in neurons that were still migrating. Although on the move, adult-born neurons were able to establish odour-evoked responses within a few hours and these responses caused large Ca 2+ transients within the cell. These findings underline a strong impact of sensory-driven activity on migrating adult-born cells right after their appearance in the glomerular layer and suggest that the path-finding process as well as the choice of their final destination might be driven by sensory stimuli. The rapid appearance of odour responsiveness found here is consistent with the data showing that immature (DPI 12–14) adult-born neurons respond to changes in odour environment with changes in their morphology and the rate of synaptogenesis [32] . Our data show that both sufficiently strong ON inputs (for sensing odourants) and odour-induced intracellular Ca 2+ signals, required for gene expression-mediated differentiation and synaptogenesis [52] , are present as early as DPI 9. Taken together, our data uncover an unexpectedly rapid appearance and maturation of odour-evoked responses in adult-born JGNs in the OB and show that sensory-driven activity is in a position to orchestrate their migration, differentiation and synapse formation, as well as their decision of when and where to integrate. Mouse preparation All experimental procedures were performed in accordance with institutional animal welfare guidelines and were approved by the government of Baden-Württemberg, Germany. The sample size of each experiment was predetermined based on biometric considerations. Two- to 6-month-old C57/BL6 mice of either sex were used in this study. All animals were randomly assigned to experimental groups, blinding was not applied. For surgery, the mice were anaesthetized with an i.p. injection of ketamine/xylazine (80/4 μg per g of body weight (BW)). Anaesthetic depth was monitored by toe pinch. Additional ketamine/xylazine (40/2 μg per g of BW) was injected when necessary. In experiments illustrated in Fig. 4 , the mice were anaesthetized with a mixture of fentanyl (0.05 μg per g of BW), midazolam (5.0 μg per g of BW) and medetomidine (0.5 μg per g of BW). After the recording chamber was glued to the skull [53] , a rectangular craniotomy (~1.2 mm × 0.7 mm) was made to expose one OB hemisphere. To reduce the movement artefacts, the dura was left intact and the craniotomy was filled with 2% agarose. Fluorescent labelling of adult-born JGNs For all experiments but the ones illustrated in Fig. 1d,e (left) and Supplementary Fig. 5 , we used a retroviral vector encoding eGFP under the cytomegalovirus immediate early enhancer-chicken β-actin hybrid promoter [54] . The complementary DNA encoding Twitch-2B biosensor ( Fig. 1d,e (left)) was also cloned into this vector in replacement of eGFP. Please note that the Twitch-2B biosensor contains brighter variants of CFP and YFP mCerulean3 and cpVenus CD . Viral injections were performed as described previously [5] . The virus-containing solution (≤1 μl) was stereotactically injected into the RMS of 2-month-old mice. Coordinates for RMS injection were 3.0 mm anterior, 0.82 mm lateral from the bregma and 2.9 mm ventral from the dura. A lentiviral vector encoding for Twitch-2B (see below) was used to generate the data shown in Supplementary Fig. 5 and was injected into the RMS using the same coordinates. The HIV-based lentiviral vector (FUGW as the backbone, Addgene 14883) containing the Twitch-2B biosensor was produced through transfection of HEK293T cells (Thermo Fisher Scientific Inc., Waltham, MA) in 10 cm plates. After 48 h, the virus-containing culture supernatant was collected, filtered through a 0.45-μm pore-sized filter and concentrated by centrifugation at 120,000 g for 2 h at 4 °C. Pellets were resuspended in PBS and stored at −80 °C. Virus-containing solutions with titre higher than 10 8 colony forming units per ml were used in this study. Chronic cranial window implantation For experiments described in Fig. 2f,g and Supplementary Fig. 2 , we implanted a chronic window over the OB of 2-month-old male mice [41] , [55] . For surgery, mice were anaesthetized with ketamine/xylazine (80/4 μg per g BW). Dexamethasone (2 μg per g BW) was administered i.p. before the surgery and lidocaine was applied locally onto the skin. Anaesthetic depth was monitored by toe pinch throughout the surgery and additional ketamine/xylazine (40/2 μg per g of BW) was injected when necessary. The skull covering both OBs was cleaned and dried. A single round opening (3 mm in diameter) was made with a dental drill and the skull overlying both OBs was carefully removed, leaving the dura intact. The surface of the dura was rinsed with sterile standard extracellular solution (composition see below) and covered with a 3-mm round coverslip (Warner Instruments, Hamden, CT). The margin between the glass and the skull was sealed with cyanoacrylic glue. The remaining exposed area over the OBs was covered with dental cement, with a small well around the coverslip. Postoperative care included an analgesic dose of carprofen (5 μg per g BW) for 3 days subcutaneously and the antibiotic baytril (Bayer, Leverkusen, Germany; 1:100 v/v) in drinking water for 10 days. After the surgery, animals were allowed to recover for 3 weeks and were subsequently examined for window clarity and new bone growth. Those mice that passed the quality control were used for eGFP virus injections into RMS, as described above. The screw housing was then affixed to the skull between the ears and was used for head fixation during consecutive imaging sessions (see below). In vivo imaging and data analysis In acute experiments, the head-attached chamber was fixed on a X – Y microscope stage and perfused with standard extracellular solution of following composition (in mM): 125 NaCl, 4.5 KCl, 26 NaHCO 3 , 1.25 NaH 2 PO 4 , 2 CaCl 2 , 1 MgCl 2 and 20 glucose, pH 7.4, bubbled with 95% O 2 and 5% CO 2 , warmed to 38 °C. The AMPA receptor blocker CNQX (6-Cyano-7-nitroquinoxaline-2,3-dione; Sigma-Aldrich, St Louis, MO) and/or NMDA receptor blocker CGP-37849 ((E,2R)-2-amino-4-methyl-5-phosphonopent-3-enoic acid; Abcam Biochemicals, Cambridge, UK; this substance is 7 fold more potent than a commonly used NMDA receptor blocker D-APV [56] ) were added to this extracellular solution. Glutamate ( Supplementary Fig. 3 ) was applied iontophoretically (MVCS-C-01M-45 unit; NPI Electronic, Tamm, Germany) directly to the cells of interest. Iontophoretic pipettes (pipette resistance 10–15 MΩ) contained 100 mM Na + -Glutamate, 10 mM HEPES, pH 7.3. To visualize the area subjected to the iontophoretic drug application, 50 μM Alexa Fluor 594 was added to the pipette solution. The animal breathed freely throughout the experiment. The respiration rate was monitored using a pressure sensor attached to the body of an animal (ADInstruments, Spechbach, Germany) and varied between 140 and 180 cycles per minute. The rectal temperature was kept at ~37 °C. The area under the craniotomy was stained with Fura-PE3 AM (TEFLAB, Austin, TX) by means of the multi-cell bolus-loading technique as described previously [38] . Imaging was performed with a customized two-photon microscope based on an Olympus FV1000 system (Olympus, Tokyo, Japan) and a MaiTai Deep See Laser (Spectra Physics, Mountain View, CA). The emitted light was collected either with a Nikon × 40 water-immersion objective (numerical aperture (NA) 0.8) or Zeiss × 20 water-immersion objective (NA 1.00). The emission of eGFP and Fura-PE3 was separated by using different excitation wavelengths of 930 and 800 nm, respectively [57] . For imaging cells labelled with the genetically encoded indicator Twitch-2B, we used 860 nm excitation light. The fluorescence emitted by the sensor was split with a 515 LP dichroic mirror and two filters: a 475/64 band-pass filter and a 500LP (Semrock, Rochester, NY) for cyan fluorescent protein and yellow fluorescent protein channels, respectively. Images were collected at 7–20 Hz (depending on the size of the imaging frame). For chronic imaging of adult-born JGNs ( Fig. 2f, g and Supplementary Fig. 2 ), the head of the mouse was fixed through the screw housing to the X – Y table, allowing reproducibility in the directions of pitch and roll. Imaging sessions were repeated every 12 h and lasted about 2 h each. For an easy identification of the field of view recorded in a previous imaging session, the blood vessels were transiently stained with sulforhodamine B (Sigma-Aldrich). The dye (1 mM), dissolved in PBS, was injected i.p. (0.1 ml per 10 g of BW). With this protocol, reliable blood vessel labelling was observed for at least 2 h. Thereafter, the staining decayed to below the detection threshold. The emission signals of eGFP and sulforhodamine B were split by a 570-nm dichroic mirror. We repeatedly imaged 13 fields of view (636 μm × 636 μm each, depth from dura up to 200 μm) from 3 mice. The eGFP-positive cells found up to a depth of 100 μm under the dura were counted and considered adult-born JGNs. The cell was counted as a migrating cell at DPI 9 if we either did not find it at DPI 10 (24 h later) or the displacement from the original position was larger than the diameter of its soma. ImageJ software ( http://rsb.info.nih.gov/ij/ ) was used to calculate the distance d between the two positions as follows: where ( x0 , y0 , z0 ) and ( x1 , y1 , z1 ) are coordinates of the target cell position measured at DPI 9 and DPI 10, respectively. For each field of view, the coordinates of the cells were set with reference to the surrounding blood vessels. Odour-responsive cells were identified using the Frame Subtraction procedure of NeuroPlex software (RedShirtImaging LLC, Decatur, GA) as described earlier [39] . Briefly, 10–20 consecutive frames (1–2 s in actual duration) corresponding to the peak of odour-evoked calcium responses were averaged and subtracted from an image obtained by averaging the same number of frames recorded immediately before the presentation of an odourant. The frame subtraction image was processed with a spatial low-pass filter that replaced each pixel with the mean of a 3 × 3 pixel region surrounding the pixel. The resulting subtracted image highlights the pixels showing a change in fluorescence in response to an odourant (for example, Figs 1c and 2b ). To exclude possible contribution of glial cells, for analyses we only used cells responding to odourant application either with firing of APs or with odour-evoked Ca 2+ transients of large amplitude (≥15% Δ F / F [39] ). Loose-seal cell-attached recordings in vivo Loose-seal cell-attached recordings were performed using an EPC-10 patch clamp amplifier (HEKA, Lamprecht, Germany) as described in ref. 39 . The recording pipettes had a resistance of 3–5 MΩ when filled with a pipette solution containing (in mM): 150 NaCl, 4.5 KCl, 10 HEPES, 2 CaCl 2 , 1 MgCl 2 , 0.05 Alexa Fluor 594, pH 7.4. To assure that we indeed record from eGFP + cells, we only accepted experiments in which a small invagination of the eGFP-labelled cytosol (green) was clearly seen within the tip of the recording pipette (red). The data were filtered at 3 kHz and digitized at 50 kHz. For spike phase and frequency analysis, we used software written in IDL (Exelis Visual Information Solutions Inc., Boulder, CO) and NeuroMatic ( www.neuromatic.thinkrandom.com/ ). For all experimental conditions, the spike frequency is given as recorded. No correction for the background spiking was performed. To test whether the spikes of a cell are locked to the respiration cycle, we made use of vector averaging. Respiration cycles were determined so that the onset of inhalation and exhalation were given phase angles θ =0° and 180°, respectively, and their intervals were linearly interpolated. For each spike of a cell, a vector with a radial coordinate r =1 and a phase angle (that is, azimuth) θ was defined in a polar coordinate system. Spikes recorded during the odourant application and those recorded before or after were analysed separately. We then obtained the vector average of respective spike vectors. The amplitude of the average vector ranged from 0 to 1 and approached 0 when the distribution of θ was random or approached 1 when all spikes were at the same phase angle. All cells analysed in the present study had average vector amplitudes of 0.12–0.33 or 0.62–0.91 ( n =20). The firing of cells was considered phase locked when the average vector amplitude was >0.62. Odourant delivery Odourants were applied through a custom-made flow-dilution olfactometer positioned in front of the snout of freely breathing mice as described previously [39] , [58] . An individual trial consisted of either one or three pulses of odourant. When thee odourant applications were used, they were applied with an interval of 14 s. The typical duration of odourant pulses was 2 or 4 s. The individual trials were separated by at least 2 min. For those experiments in which response amplitude had to remain stable over an extended period of time (for example, wash in and wash out of the NMDA receptor blocker CGP-37849), the interval between the trials was increased to 10 min. To identify odourants that activated the cell of interest, we tested three to five odourants known to evoke activity in dorsal glomeruli [59] , [60] , [61] . The most commonly used were 2-hexanone, isoamyl acetate, hexanal, benzaldehyde and ethyl tiglate. To obtain the data shown in Fig. 1d,e (left panel), adult-born cells were stimulated with a mixture of three odourants (2-hexanone, isoamyl acetate and ethyl tiglate; 0.6% of saturated vapour each). All the odourants were purchased from Sigma-Aldrich and of highest commercially available purity. Adult-born cells were considered non-responding if they failed to respond to the odourant activating their parent glomerulus at the highest concentration tested (that is, 9% of saturated vapour). Immunohistochemistry After decapitation, brains were removed and fixed with 4% formaldehyde in PBS for 24 h at 4 °C. Next, the brains were cryoprotected in PBS containing 25% sucrose (overnight, at 4 °C), followed by embedding in Tissue Tek (Sakura, Zoeterwoude, The Netherlands) and freezing at −80 °C. The antibody labelling was performed on free-floating horizontal cryoslices (40–50 μm thick) at room temperature. To prevent nonspecific background staining, the sections were treated with a blocking solution (5% normal donkey serum and 1% Triton X-100 in PBS) for 1 h. After blocking, slices were exposed overnight to primary antibodies diluted in blocking solution. Next, the sections were rinsed in PBS three times for 10 min and incubated with secondary antibodies diluted 1:1,000 (in PBS +2% BSA) for 2 h in the dark. For BrdU immunostaining, sections were pretreated 30 min at 37 °C with 2 N HCl in PBS containing 0.5% Triton X-100, for DNA denaturation before the treatment with the blocking solution. Finally, the sections were washed three times in PBS, transferred to Superfrost Plus charged glass slides (Langenbrink, Emmendingen, Germany) and were mounted in Vectashield Mounting Medium (Vector Laboratories, Burlingame, CA). Alternatively, ProLong Gold Mounting Medium (Invitrogen, Grand Island, NY) was used. The following primary antibodies were used in conjunction with the antibody against GFP (goat or rabbit anti-GFP, Rockland 600-101-215 or 600-401-215, 1:2,500 or 1:1,500): rabbit polyclonal antibody against DCX (Abcam ab18723, 1:2,000), mouse monoclonal antibody against Polysialic acid–neural cell adhesion molecule (Millipore MAB5324, 1:1,500), sheep polyclonal antibody against TH (Millipore AB1542, 1:2,000), mouse monoclonal antibody against calretinin (Swant 6B3, 1:2,000), rabbit polyclonal antibody against calbindin (Swant CB-38a, 1:4,000), rabbit polyclonal antibody against GABA transporter VGAT (Millipore AB5062P, 1:500), mouse monoclonal antibody against NeuN (Millipore MAB377, 1:500), rat monoclonal anti-BrdU antibody (Abcam ab6326, 1:200). The secondary antibodies were as follows: donkey-anti-goat or anti-rabbit IgG-conjugated Alexa Fluor 488 (A11055 or A21206, 1:1,000), donkey-anti-rabbit, anti-mouse or anti-sheep IgG-conjugated Alexa Fluor 594 (A21207/A21203/A11016, 1:1,000), donkey-anti-mouse IgG conjugated Alexa Fluor 680 (A10038, 1:1,000), all purchased from Invitrogen. Labelled slices were imaged using the Olympus Fluoview 300 laser scanning microscope coupled to a MaiTai mode-locked laser operating at 690–1,040 nm wavelength (Spectra Physics). Alexa Fluor 488 and 594 were excited simultaneously at 800 nm and their fluorescence was split with a 630LP dichroic mirror. Alexa Fluor 680 was excited at 900 nm. Cells were considered positive for a given marker, if the brightness of the cell exceeded 3 × s.d. of the noise level recorded in the nearby region of interest of the same size (that is, ‘background’ region). To analyse the distribution of VGAT-positive dots in adult-born neurons ( Fig. 6 ), we used a Zeiss LSM 710 confocal system (pinhole size 64 μm) equipped with a Zeiss × 63 oil-immersion objective (NA 1.4). The fluorophores were excited sequentially at 488 nm (Alexa Fluor 488) and 561 nm (Alexa Fluor 594), and filtered with respective single-band band-pass filters (542/44 and 660/75 nm). Quantification of the number of VGAT-positive dots was performed on stacks of eight bit confocal image planes spaced by 0.45 μm using the software ZEN 2012. We carefully examined the co-localization of eGFP and VGAT signals in all three projections for example, see Fig. 6b ) and only counted VGAT-positive dots that were located within the GFP + dendrites in all three ( x – y , y – z and x – z ) single-frame images. For experiments illustrated in Supplementary Fig. 4 , anti-DCX antibodies were visualized with Alexa Fluor 594, anti-GFP antibodies with Alexa Fluor 488 and antibodies against calbindin, calretinin, TH and NeuN were visualized with Alexa Fluor 680. This combination of antibodies was necessary, because many neurons in the glomerular layer do not express the usual marker of mature neurons NeuN [62] . After labelling, preparations were sequentially imaged at 800 nm excitation light using a 570LP dichroic mirror (thus separating fluorescence from Alexa Fluor 488 (blue in Supplementary Fig. 4 ) and Alexa Fluor 594, 630 (green in Supplementary Fig. 4 )), and at 900 nm excitation light using a 630LP dichroic mirror. As Alexa Fluor 594 is poorly excited at 900 nm, the latter imaging condition separated Alexa Fluor 488 from Alexa Fluor 680 (red in Supplementary Fig. 4 ). When merging all images together, Alexa Fluor 488 appeared blue, Alexa Fluor 594 green and Alexa Fluor 630 appeared green and red, and thus yellow ( Supplementary Fig. 4 ). Statistics Statistical analyses were performed using Igor Pro, Microsoft Office Excel 2007 and SPSS Statistics 15. We used the Shapiro-Wilk Test (Excel 2007) to test for the normality of data. Parametric tests were applied for testing the equality of means of normally distributed data sets (unless otherwise indicated, all data are shown as mean±s.e.m.). When choosing which tests to use for skewed distributions with unequal variances, we followed recommendations of Fagerland and Sandvik [63] . All the statistical tests were two sided. P -values≤0.05 were considered statistically significant. How to cite this article: Kovalchuk, Y. et al . In vivo odourant response properties of migrating adult-born neurons in the mouse olfactory bulb. Nat. Commun. 6:6349 doi: 10.1038/ncomms7349 (2015).